Understanding and controlling plasmon-induced convection The heat generation and fluid convection induced by plasmonic nanostructures is attractive for optofluidic applications. However, previously published theoretical studies predict only nanometre per second fluid velocities that are inadequate for microscale mass transport. Here we show both theoretically and experimentally that an array of plasmonic nanoantennas coupled to an optically absorptive indium-tin-oxide (ITO) substrate can generate >micrometre per second fluid convection. Crucially, the ITO distributes thermal energy created by the nanoantennas generating an order of magnitude increase in convection velocities compared with nanoantennas on a SiO 2 base layer. In addition, the plasmonic array alters absorption in the ITO, causing a deviation from Beer–Lambert absorption that results in an optimum ITO thickness for a given system. This work elucidates the role of convection in plasmonic optical trapping and particle assembly, and opens up new avenues for controlling fluid and mass transport on the micro- and nanoscale. Plasmonic systems are drawing much attention due to their broad applications in several fields such as biology [1] , sensing [2] , nanoscale heating [3] , nonlinear optics [4] , [5] , optofluidics [6] , [7] , [8] and optical trapping [9] , [10] , [11] , [12] , [13] , [14] . Indeed, light-absorbing nanotextured surfaces such as those utilizing metal pads, dipole antennas and bowtie nanoantennas have recently been shown to be very effective for optical manipulation [9] , [13] , [15] . These plasmonic ‘nanotweezers’ have multidisciplinary applications spanning biological species manipulation [16] , colloidal physics and optical matter formation [9] , [17] , DNA aggregation [15] , lab-on-a-chip particle manipulation [6] and fundamental optical physics [18] . In all cases, thermal convection generated as a result of the frequency-dependent absorption of optical energy by the metallic nanostructures plays an important role in the particle trapping behaviour observed [9] , [12] . However, recent efforts to theoretically describe the fluid convection generated in a plasmonic architecture comprising an isolated Au pad have shown only weak convection velocities, even with temperatures approaching the boiling point of water [19] . Evidently, there is a limited current understanding of how the high-velocity (μm s −1 or greater) fluid convection observed in plasmonic optical trapping is generated [6] , [9] . These flows have been shown to alter particle dynamics, giving rise to trapping phases in plasmonic nanotweezer applications [9] , and are required to make plasmonics and light absorption-based techniques in general viable for lab-on-a-chip optofluidics [6] . To this end, joining the established capabilities of plasmonic devices with the ability to effectively control fluids on the micro- and nanoscale using light can enable higher degrees of dexterity, for example, in moving analytes or objects within an on-chip environment [6] . As such, understanding the generation of high-velocity thermo-plasmonic convection (defined here as convection with velocities on the order of μm s −1 ) is both important for a complete physical picture of plasmonic optical trapping and is highly attractive across a broad range of disciplines. Here, we present theoretical and experimental results characterizing fluid convection generated via optical absorption by an array of bowtie nanoantennas (BNAs) and a base indium-tin-oxide (ITO) substrate layer. We find that the BNAs alone provide an order of magnitude increase over the 5–10 nm s −1 velocities generated by an isolated nanostructure; however, an additional order of magnitude increase can be achieved when considering the optically absorptive, ITO substrate layer. We show that the ITO layer both effectively distributes thermal energy and significantly increases the spatial extent of the temperature distribution, and is thus crucial for developing μm s −1 velocities. The thermal and convective responses of the system are investigated under several nanoantenna resonance conditions and ITO thickness values, revealing that large convection velocities can be achieved in all cases, but with reduced sensitivity for off- and near-resonant excitation. Crucially, we demonstrate that the modification of optical absorption in systems of varying ITO thickness leads to an optimum ITO thickness for achieving the highest possible convection velocities for a given system. This enables the engineering of specific thermal and fluidic responses from a given nanoantenna system. To this end, we demonstrate control of fluid velocities spanning hundreds of nm s −1 to μm s −1 by varying ITO thickness, input wavelength and input optical power. Theoretical model Thermo-plasmonic convection arises due to the electromagnetic heating in metallic nanostructures that results from dissipative losses [3] . This in turn establishes a temperature gradient and produces buoyancy-driven natural convection currents. This process is governed by a set of coupled partial differential equations describing the electromagnetic (EM), heat-transfer (HT) and fluid mechanics (FM) phenomena. We make use of a commercial software package (COMSOL Multiphysics) and start by solving the time-independent vector wave equation [20] where E is the total electric field in the vicinity of the nanostructures, k 0 =2π/ λ is the free-space wavenumber with wavelength λ , and ( r )= ′( r )− i ′′( r ) is the complex, position-dependent ( r ) permittivity with real and imaginary parts ′ and ′′, respectively. Equation (1) is then used to obtain the heat source density q ( r )=1/2Re[ J · E *] (ref. 20 ), where J is the induced-current density in each nanoantenna and the ITO, Re stands for real part and * is the complex conjugate. The optical properties of ITO vary according to specific preparation and elemental content, and therefore standard values are not established. Here, we set the dielectric function for ITO to be ′= 3.338, 3.181 and 3.096, ′′=0.2359, 0.2716 and 0.2953 for λ = 685, 785 and 860 nm, respectively, in accordance with ref. 21 ( Supplementary Fig. 1 ); the optical properties for Au are taken from Johnson and Christy [22] . The heat source density is used to find the heat power generated by each element, Q i =∫∫∫ q i ( r )d 3 r (ref. 20 ). The total heat power Q tot =∑ i Q i serves as a source term for the coupled, steady-state HT-FM problem [23] where T ( r ), u ( r ) and p ( r ) are the spatial temperature, fluid-velocity and pressure distributions, respectively, and the material parameters are k , ρ , c p and η (thermal conductivity, density, heat capacity and kinematic viscosity, respectively). For ITO, ρ = 7,150 kg m −3 , c p =340 J kg −1 K −1 and κ =10.2 W m −1 K −1 (ref. 24 ). The Boussinesq approximation is used and the buoyancy-driven natural convection is described via an imposed volume force, F = gρ 0 β ( T ) [ T ( r )− T 0 ] , where g is gravitational acceleration, ρ 0 =998 kg m −3 and T 0 =20 °C are the reference density of water and temperature, respectively, and β ( T ) is the temperature-dependent thermal expansion coefficient of water. The geometry of the problem is depicted in Fig. 1 . 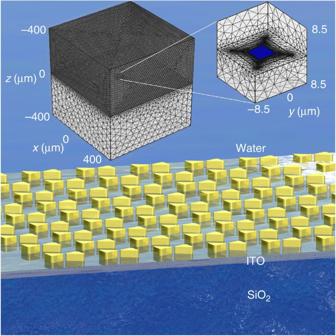Figure 1: Geometry for the simulation. A 9 × 9 array of Au bowtie nanoantennas is placed on an ITO square embedded in a thick SiO2substrate and immersed in water. The inset shows the meshed domain with representative dimensions. Figure 1: Geometry for the simulation. A 9 × 9 array of Au bowtie nanoantennas is placed on an ITO square embedded in a thick SiO 2 substrate and immersed in water. The inset shows the meshed domain with representative dimensions. Full size image The EM problem is solved for a 9 × 9 rectangular array of Au BNAs, separated by a gap-to-gap spacing of Γ=425 nm. Individual bowties have a 120-nm altitude, 15-nm tip radius of curvature, 50-nm thickness and 20-nm gap. The BNAs are placed on 50, 75 or 100-nm thick ITO square with 15-μm side length that is embedded in a 8.5-μm thick SiO 2 substrate. The system is immersed in water and illuminated substrate-side first by a laser with a Gaussian intensity distribution and focal-spot radius w 0 =0.61 λ /NA, where NA=0.6 is the numerical aperture of the focusing objective lens. The input Gaussian beam is polarized parallel to the bowtie tip-to-tip axis. Further, we do not consider vectorial focusing behaviour for the lens due to the relatively low NA; the axial polarization component contributes <5% of the total intensity at focus [25] . Three wavelengths λ OR , λ NR and λ R (off-resonant, near-resonant and resonant) corresponding to 685, 785 and 860 nm, respectively, are used in the simulation. Unless otherwise noted, a maximum power of 5 mW is used. 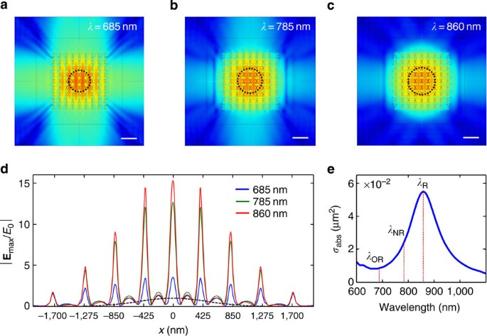Figure 2: Simulated EM results. Spatial field distributions for (a) off-resonant, (b) near-resonant and (c) resonant illumination; scale bars are 1 μm. (d) Field distribution line plot showing a horizontal cut through the middle of the array; dashed lines indicate the focal spot of the Gaussian beam. (e) Plot of the spectral absorption cross section of the BNAs. Electromagnetic response Figure 2 shows the 2D electric field spatial distributions | E / E 0 |, where E 0 is the electric field amplitude of the input Gaussian beam and | E |= , along with a 1-D line plot taken horizontally through the centre of the BNAs. The resonance of this system is evident from the spectral absorption cross section σ abs =−∫∫1/2Re[ E × H *]·d S / I 0 , where E and H are the total electric and magnetic fields inside a rectangular surface with area element d S that encloses one unit cell of the array and I 0 is the incident intensity. Figure 2: Simulated EM results. Spatial field distributions for ( a ) off-resonant, ( b ) near-resonant and ( c ) resonant illumination; scale bars are 1 μm. ( d ) Field distribution line plot showing a horizontal cut through the middle of the array; dashed lines indicate the focal spot of the Gaussian beam. ( e ) Plot of the spectral absorption cross section of the BNAs. Full size image The EM response of the array results in excitation of antennas outside of the 0.6 NA Gaussian focal spot (indicated by dotted black lines) for all resonance conditions. This effect arises from the near-field diffraction of the incident light by the grating formed by the nanoantenna array [26] , [27] , [28] , [29] . When the incident light matches the critical grating period Γ c = mλ 0 /( n ITO sin θ inc + ), where m =1 is the diffraction order, n ITO is the refractive index of the ITO (water) and θ inc is the incident angle, incident light switches from evanescent to propagating, is diffracted parallel to the transverse plane, and results in a grating resonance, also known as the Rayleigh anomaly [26] , [28] . Here, Γ c ~515, 590 and 650 nm for λ OR , λ NR and λ R , respectively. Thus, increasing the incident wavelength from 685 to 860 nm corresponds to a red-detuning from Γ=425 nm. Given that Γ<Γ c , the grating order is evanescent, however, it still causes near-field interactions between the bowties that are increasingly suppressed with increasing wavelength [30] ; this effect is evident in the spatial field distributions, which show diffracted side lobes that decrease in intensity with increasing wavelength. In addition, the diffractive excitation of nanonantennas outside of the focal spot can be seen from the field distribution line plots, which exhibit field-enhancement peaks occurring at integer multiples of the grating period Γ (at the location of the bowties). Outside of the central 3 × 3 bowties, there is a vanishingly small input field; however, the outer bowties display strong enhancement peaks. As a result, each element in the extended array participates in the fluid convection process by a collaborative heating effect. Heating and induced fluid convection A vertical 2D slice of convection velocity profile overlaid on the temperature distribution, defined as Δ T = T ( r )− T 0 is shown in Fig. 3a . We see that convection pattern, which is nearly radially symmetric, indeed possesses the features of a toroidal Rayleigh–Bénard flow; this is likely the reason that thermo-plasmonic convection has been mistakenly referred to as Rayleigh–Bénard flows in the literature. However, Rayleigh–Bénard convection arises from an instability in a channel with a uniformly heated bottom surface when the Rayleigh number, Ra= ρ 0 βg Δ Tℓ 3 /( ηα ), where ℓ is the characteristic length of the system and α = κ /( ρ 0 c p ) is the thermal diffusivity, exceeds a critical value ~1,700 (ref. 31 ). Such a system is quiescent until Δ T across the entire fluid cell is large enough to cause the instability. Whereas the spatially nonuniform heating in plasmonic systems generates fluid convection at any finite Rayleigh number Ra>0 and is not associated with instability. 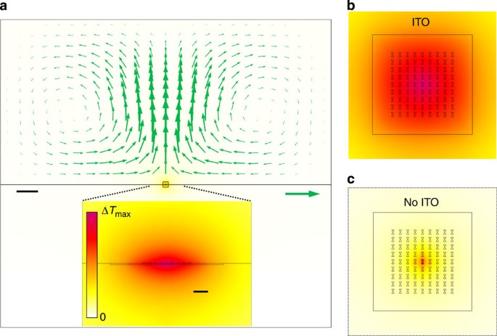Figure 3: Simulated HT-FM results. (a) Fluid convection pattern overlaid on the temperature distribution generated by resonant illumination of the BNAs+ITO system. The included green reference arrow indicates 1-μm s−1fluid velocity and the (left-hand) scale bar is 50 μm. The inset shows the temperature distribution near the BNAs and the inset scale bar is 1 μm. (b) ‘Top’ view of the temperature distribution of the BNAs with a 75-nm thick ITO slab. (c) Temperature distribution of the BNAs without an ITO slab; black dotted lines showing the edge of the temperature distribution are included for clarity. Figure 3: Simulated HT-FM results. ( a ) Fluid convection pattern overlaid on the temperature distribution generated by resonant illumination of the BNAs+ITO system. The included green reference arrow indicates 1-μm s −1 fluid velocity and the (left-hand) scale bar is 50 μm. The inset shows the temperature distribution near the BNAs and the inset scale bar is 1 μm. ( b ) ‘Top’ view of the temperature distribution of the BNAs with a 75-nm thick ITO slab. ( c ) Temperature distribution of the BNAs without an ITO slab; black dotted lines showing the edge of the temperature distribution are included for clarity. Full size image The temperature distribution in the array is strongly dependent on the presence of ITO as evidenced in the ‘top down’ view in Fig. 3 , which depicts BNAs under resonant illumination with ITO and without ITO, Fig. 3b,c , respectively; the temperature distributions are plotted with the same temperature range. We note that aside from peak temperatures, there are only slight variations in the temperature distributions for the various resonance conditions for a given system. Clearly, the ITO significantly increases the spatial extent of the temperature distribution compared with BNAs on bare SiO 2 . The mechanism for this is two fold. First, the thermal conductivity of ITO is ~10 times higher than that of SiO 2 , and therefore the heat generated by the nanoantennas can more easily diffuse throughout the ITO substrate. Second, since ITO is also intrinsically absorptive, it generates endogenous heat power via dissipative losses, which in turn increases the temperature and heat flux in the areas between individual nanoantennas. Since ITO (or similar materials) are present in many plasmonic systems, its effect on heating and temperature distributions is an essential component for characterizing thermo-plasmonic convection. Given that the buoyancy force is dependent on the spatial temperature distribution, the presence of the ITO strongly influences the maximum convection velocities achieved in the system. We note that, for all parameters in this study, the steady-state velocity distributions appear nearly identical with the only difference being the maximum velocity achieved for the given parameter set. The effect of including the ITO substrate is evident in Fig. 4a —the maximum velocities of 750, 1,310 and 1,325 nm s −1 for λ OR , λ NR and λ R , respectively, are at least one order of magnitude larger than those attained using an SiO 2 substrate instead of the ITO. However, the increased fluid velocities when using ITO compared with a bare SiO 2 substrate may lead to decreased controllability of the fluid flow in the former case. For BNAs without ITO, v max does not exceed 200 nm s −1 despite Δ T max >40 °C. This can be attributed to the fact that the low thermal conductivity of the SiO 2 substrate causes the temperature distribution to be concentrated near the central illumination spot, as shown in Fig. 3 . This prevents effective transduction of the thermal energy to the fluid bath, thereby leading to lower overall fluid velocities despite a substantial temperature increase. In contrast, the dissipative heating from a 10 × 10 μm 2 ITO slab alone establishes convection currents approaching 300 nm s −1 with a 20 °C increase for the 5 mW input power. Compared with an isolated bowtie on SiO 2 , the BNAs produce an order of magnitude increase in convection velocities. However, simply placing the antennas in an array is insufficient to generate μm s −1 fluid velocities, as assumed in previous studies. These results clearly demonstrate the importance of the ITO substrate for maximizing convection velocities for a given nanonantenna system. 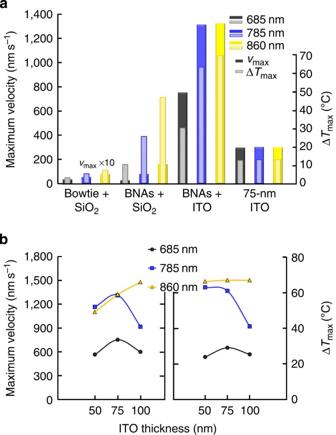Figure 4: System comparison and ITO screening. (a) Maximum fluid velocity and temperature increase for the various systems. When present, ITO thickness is 75 nm. Solid (striped) bars correspond to velocity (temperature). Fluid velocities for the bowtie with SiO2case are scaled 10 × for clarity. (b) Velocities and temperatures as a function of ITO thickness for all three resonance conditions considered. Solid lines are included to guide the eye. Figure 4: System comparison and ITO screening. ( a ) Maximum fluid velocity and temperature increase for the various systems. When present, ITO thickness is 75 nm. Solid (striped) bars correspond to velocity (temperature). Fluid velocities for the bowtie with SiO 2 case are scaled 10 × for clarity. ( b ) Velocities and temperatures as a function of ITO thickness for all three resonance conditions considered. Solid lines are included to guide the eye. Full size image Figure 4b shows the velocity and temperature increase calculated as a function of ITO thickness. For all cases, increasing the thickness of ITO ( t ITO ) from 50 to 75 nm produces larger velocities and temperatures due to a larger volumetric heat production by the substrate. For thicknesses above this point for λ OR and λ NR , the ITO screens the BNAs from the excitation light, effectively reducing their optical absorption, and thus drives down the maximum temperature and velocity developed by the system. However, for resonant illumination the increase in v max above 75-nm ITO can be attributed to the fact that the absorption cross section at λ R is at least two times that of the off-resonant cases. Thus, the enhanced absorption by the resonant BNAs can offset the input-wave attenuation from the 100-nm thick ITO. This is supported by the fact that the maximum temperature remains approximately the same after a 33% increase in t ITO . The behaviour of v max and Δ T max as a function of t ITO indicates that the absorption in the system does not follow a simple Beer’s law form, wherein the intensity after the ITO (the BNA excitation intensity) is given by I = , where γ is the absorption coefficient of the ITO [32] . In this picture, increasing t ITO enhances volumetric absorption and therefore Q ITO , the heat generation in the ITO, which would drive the temperature of the system upwards. For ITO without BNAs, this monotonic increase of Q ITO with t ITO is indeed observed. However, for BNAs with ITO, we find that the heat power dissipated in the ITO for λ OR ( λ NR ) decreases from 120 μW (190 μW) to 90 μW (160 μW) as t ITO increases from 75 to 100 nm. This suggests that the presence of the BNAs modifies the heat absorption in the ITO from the nominal case of ITO alone, and thus gives rise to the nonlinear behaviour observed in Fig. 4b . The novel, nanoantenna-mediated absorption in the ITO substrate may be useful for independent control of thermo-plasmonic fluid convection velocities and temperature. Furthermore, this has important implications for plasmonic optical trapping, where particle dynamics are dependent on the local temperature and induced fluid velocities. Experimental measurement of plasmon-induced convection To verify the effect of the ITO on the thermo-fluidic response of the BNAs, we measure the convection velocity of polystyrene tracer particles for h ITO = 50, 75 and 100 nm and input wavelengths λ = 685, 785, and 860 nm; the results are summarized in Fig. 5 . The power at the focal plane is set to 2.5 mW for all cases due to experimental limits in available power at λ =860 nm. Given that v max and Δ T max scale linearly with input power over the entire range of Δ T =0 to the boiling point of water ( Supplementary Figs 2 and 3 ), the trends in v max and Δ T max as a function of h ITO should be preserved when using lower input power, compared with those observed theoretically in Fig. 4 . The ITO screening effect is evident in Fig. 5a , which shows the measured convection velocities for the BNAs+ITO system. Here, velocities are maximized at h ITO =75 nm and decrease with increased ITO thickness for all three resonance conditions. To rule out the possibility that anomalously large absorption in the 75-nm ITO sample causes the observed maximum, we measured convection velocities on an ITO-only system under the same input optical conditions. 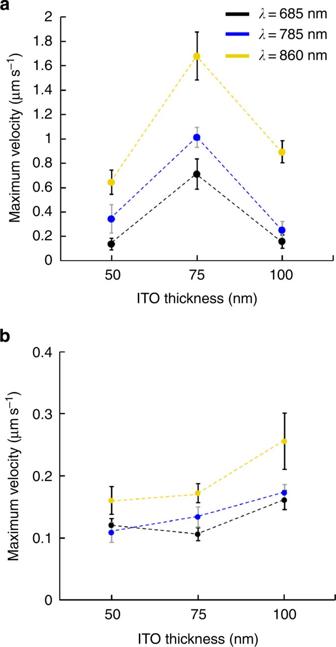Figure 5: Experimental convection results. Measured convection velocities for the (a) BNAs+ITO system and (b) the ITO-only system. Black, blue and gold data points correspond toλOR,λNRandλR, respectively. Error bars represent the standard error in the velocity measurement over 10 experimental runs for each data point, and grey error bars are used forλNRdata for clarity. Dashed lines are included to guide the eye. Figure 5b shows that for all resonance conditions, the maximum velocities occur at h ITO =100 nm, which is consistent with standard Beer–Lambert absorption in the ITO-only system. This further supports that ITO screening and deviation from the Beer–Lambert model are responsible for the observed maximum in Fig. 5a . The fact that ITO screening is observed for λ R indicates that the effect is stronger than theoretically predicted. In addition, measured velocities are larger than predicted values for all three resonance conditions. Taken together, these observations suggest that the absorption by the ITO substrate is stronger than theoretically predicted. Figure 5: Experimental convection results. Measured convection velocities for the ( a ) BNAs+ITO system and ( b ) the ITO-only system. Black, blue and gold data points correspond to λ OR , λ NR and λ R , respectively. Error bars represent the standard error in the velocity measurement over 10 experimental runs for each data point, and grey error bars are used for λ NR data for clarity. Dashed lines are included to guide the eye. Full size image The discrepancies between measured and predicted results can be attributed to several factors. First, inevitable variation in the processing environment of each sample can result in slight geometrical and material modifications that can affect the optical response. Furthermore, the deviation of the optical properties of the ITO films compared with modelled values can contribute to the larger velocities and increased screening observed. Second, the Au nanoparticles are polycrystalline in nature, which results in larger heat generation and therefore larger convection velocities compared with the modelled single-crystalline structures [33] . Notwithstanding the differences between experimental and theoretical results, the data clearly show that h ITO is a critical parameter that can be used to tailor the performance of thermo-plasmonic convection, thereby offering an effective route to control fluid and particle motion in plasmonic systems. The results of our computational model are further verified by using time-lapse video microscopy to observe the convection velocities of 1–20 μm-diameter, PMMA tracer particles placed in BNAs+ITO ( Supplementary Movie 1 ) and ITO-only systems ( Supplementary Movie 2 ). Movies are taken with a frame rate of 0.2 frames per second for several minutes to compute the average convection velocities of the particles. 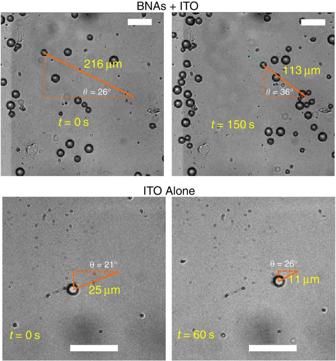Figure 6: Time-lapse convection frames. Experimental demonstration of fluid convection in the coupled BNA+ITO system (top panels) and the ITO alone (bottom panels). Scale bars in the top (bottom) panels correspond to 50 μm (25 μm). Figure 6 provides direct experimental evidence of the high-velocity, large-scale fluid convection produced by our system. The orange line connects the centre of the particle of interest with the location of the focal spot. For BNAs+ITO, we see average particle convection velocities ranging from ~600 to 900 nm s −1 , which is in fair agreement with the model; the ITO film alone produces convection velocities of ~200 nm s −1 , which corresponds well with the values predicted by the model. The angles of the particle trajectory are provided to show that particles are drawn towards the focal spot in a radial manner. As particles approach the optical axis, optical forces can contribute significantly to the particle dynamics. In particular, we observe rapid acceleration of particles in the transverse plane and strong axial ‘scattering’ away from substrate once they approach within ~5 μm of the focal spot ( Supplementary Movie 3 ). However, within this region, it is difficult to experimentally separate the individual contributions of optical and other forces. As a result, convection velocities are determined by investigating particle motion in a region >10 μm outside of the focal spot, where optical forces and thermophoresis do not contribute to particle motion. To the best of our knowledge, this work represents the first demonstration of convection using only thin ITO layers, a feature that opens an avenue for future investigations of light-driven mass transport in nonplasmonic-based optofluidic systems. Figure 6: Time-lapse convection frames. Experimental demonstration of fluid convection in the coupled BNA+ITO system (top panels) and the ITO alone (bottom panels). Scale bars in the top (bottom) panels correspond to 50 μm (25 μm). Full size image The linearity of v max and Δ T max is expected due to the small contribution of the (nonlinear) first term in Equation 3. Comparing different systems by fitting these data to a linear curve, we can extract δ v and δ T slope parameters that can be regarded as velocity and temperature ‘sensitivity’ values for each combination of wavelength and ITO thickness in that they characterize the respective responses for a unit power change ( Supplementary Fig. 2 ). It is seen that the off-resonant illumination results in a lower sensitivity of the plasmonic convection velocity and temperature to a unit increase of input power. As a result, λ OR should be utilized with higher input powers than λ NR and λ R and may be useful in applications including particle trapping, nonlinear optics and sensing [11] . The sensitivity at each wavelength as a function of ITO thickness follows the same behaviour as observed in Fig. 4 . Specifically, the sensitivity for λ R increases monotonically with t ITO , whereas for λ OR and λ NR it displays a maximum near 75 nm. Given that δ v ( t ITO ) and δ T ( t ITO ) are derived from the system response over a range of input powers, these quantities serve as useful design parameters for a given plasmonic convection system. The collaborative effect of nanoplasmonic arrays has been previously shown to shift the peak resonance and increase the field enhancement properties of individual antennas [5] , [29] ; however, few studies have explored the heating effects of such arrays. To this end, our work provides insight into the physics of plasmonic arrays by showing that diffractive effects enable elements outside of the excited region of the input field to participate in the heating process, thereby increasing maximum temperature and enhancing fluid velocities [26] . The experimental observation of these convection velocities are in fair agreement with theoretical predictions; however, discrepancies exist due, in part, to differences in the optical properties of the actual and simulated ITO films and the polycrystalline nature of the structures. Specifically, it is well-established that ITO films and Au nanostructures prepared via e-beam lithography and evaporation are polycrystalline in nature [34] . Compared with the homogeneous structures simulated in this study, the polycrystalline structure of ITO and Au that could be an additional source of deviation from the model in practice. We performed comparable simulations using a 0.25 NA lens, which produces a larger focal spot, and find that the only difference from the results for 0.6 NA is lower δ v and δ T values ( Supplementary Fig. 3 ). Finally, while optical forces clearly contribute to the particle motion near the optical axis, calculation of these forces on the 1–10-μm diameter particles via Maxwell stress tensor methods requires extremely fine mesh elements over the entire 17-μm 3 computational domain [10] . This poses a considerable computational challenge and will be the subject of a future study. We have shown that when utilized with an optically absorptive substrate, plasmonic arrays can effectively produce high-velocity (>1 μm s −1 ) convection currents spanning hundreds of microns with frequency-tunable sensitivities. We find that the presence of BNAs alters the absorption in the ITO, thereby indicating an optimum ITO thickness for attaining maximum convection velocities and temperature. This behaviour is useful for tuning the thermal and convective responses, thereby enabling control of fluid velocities spanning several orders of magnitude. The methods for achieving (frequency-tunable) rapid convection outlined in this work, that is, using nanoantenna arrays in conjunction with an absorptive substrate, can be used in optofluidic applications for solar energy collection, photobioreactors and photochemistry [35] . Plasmonic devices are especially useful for applications where low-input power is required (for example, collecting and manipulating biological species), yet significant fluid motion is desired. Furthermore, the bare ITO substrate can achieve similar effects with reduced fabrication costs, at the expense of increased optical power requirements, and therefore is attractive for lab-on-a-chip technologies that do not rely on the use of plasmonics. These results have important implications for explaining previously observed dynamics in plasmonic nanotweezers including self-assembly of large particle clusters [9] . The theoretical prediction and experimental demonstration of both plasmonic and ITO-induced convection in this work will be useful for the growing range of disciplines that utilize plasmonic devices and could open new avenues for controlling fluid flow on the micro- and nanoscale. Solution method We make use of a commercial solver (COMSOL Multiphysics) for the simulations. The full-EM domain is a 17 × 17 × 17 μm cube, and ‘scattering’ boundary conditions (BCs) are used on all outer boundaries; this BC allows EM radiation to propagate out of the simulation domain without reflection. The symmetry of the system allows for perfect electric and perfect magnetic conductor BCs to be placed along the x and y axes, respectively, thereby reducing the domain by 4 × for only the EM computation. Subsequently, the full EM domain is placed inside a larger 800 × 800 × 800 μm 3 domain for the HT-FM computation (see inset in Fig. 1 ). Each boundary of the HT-FM domain is set with a no-slip wall condition, that is, u =0 at each boundary [23] and a prescribed temperature of T 0 . The EM problem uses ~10 6 mesh elements and 30 GB RAM, and the HT-FM problem is meshed with an additional 5 × 10 5 elements, using ~45 GB RAM total. The relative error residual for convergence is set to 10 −3 for all calculations; reducing the tolerance further to 10 −4 and 10 −6 has no effect on the returned solution. Fabrication The BNAs are patterned by electron beam lithography (EBL) on ITO-coated SiO 2 substrates using a JOEL EBL system. To produce varying ITO thickness, a Cooke Dual-Gun sputtering system is used with 8 sccm flow of Argon gas at 2 × 10 −6 torr of pressure. Calibration of the ~9 nm min −1 deposition rate is performed by a Metricon Model 2010/M Prism Coupler and KLA-Tencor Alpha-Step IQ profilometer. For the BNAs, a 100-nm thick PMMA e-beam resists layer is spun on the substrate and baked at 200 °C for 2 min. After exposure, the resist is developed in IPA:MIBK 3:1 for 45 s, rinsed with isopropyl alcohol for 30 s and dried under a stream of high-purity nitrogen. Using a dual-gun electron-beam evaporation chamber, a 3-nm thick Cr adhesion layer followed by a 50-nm thick Au layer is deposited. Metal lift-off is performed by soaking the sample in acetone for 30 min. Experimental A standard brightfield microscope is used to monitor the trajectory of 6-μm diameter polystyrene particles as a result of thermo-plasmonic heating; this particle size is chosen to minimize the influence of Brownian motion. The 785- and 860-nm excitation is derived from a Ti:sapphire laser (Spectra Physics Mai Tai) operated in a continuous-wave mode. The 685-nm source is derived from a custom diode laser assembly with a spatial filter to ensure a Gaussian profile. Care is taken to produce an identical beam diameter for the two sources at the input of the 0.6-NA objective. Time-lapse video microscopy (0.2 Hz frame-rate) is utilized to monitor the trajectory of particles approaching to within ~10 μm of the focal spot; this ensures no influence of optical forces on average particle velocity. Velocity data are recorded for 10 individual particles, for each combination of ITO thickness and wavelength, by tracking the centroid of the particle as it approaches from ~50 μm to within 10 μm of the focal spot. Error bars correspond to standard error for the velocity measurements. How to cite this article: Roxworthy, B. J. et al . Understanding and controlling plasmon-induced convection. Nat. Commun. 5:3173 doi: 10.1038/ncomms4173 (2014).